Transferring a synthetic gene circuit from yeast to mammalian cells The emerging field of synthetic biology builds gene circuits for scientific, industrial and therapeutic needs. Adaptability of synthetic gene circuits across different organisms could enable a synthetic biology pipeline, where circuits are designed in silico , characterized in microbes and reimplemented in mammalian settings for practical usage. However, the processes affecting gene circuit adaptability have not been systematically investigated. Here we construct a mammalian version of a negative feedback-based ‘linearizer’ gene circuit previously developed in yeast. The first naïve mammalian prototype was non-functional, but a computational model suggested that we could recover function by improving gene expression and protein localization. After rationally developing and combining new parts as the model suggested, we regained function and could tune target gene expression in human cells linearly and precisely as in yeast. The steps we have taken should be generally relevant for transferring any gene circuit from yeast into mammalian cells. The emerging field of synthetic biology applies engineering principles to design and build biological systems for predefined purposes [1] , [2] . Promising applications such as biofuel production [3] and drug synthesis [4] have stimulated rapid advances in this field. To date, most progress has occurred in microorganisms [5] , [6] , [7] , [8] , [9] , [10] , [11] , while mammalian synthetic biology has lagged behind. Synthetic mammalian constructs, including inducible gene expression systems [12] , [13] , [14] , logic gates [15] , [16] , memory devices [17] , [18] and genetic oscillators [19] have employed molecular machinery specific to higher eukaryotes [20] , [21] . While these examples suggest that similar functions could be achieved in microbes and mammalian cells, the principles and methodology of gene circuit transfer into mammalian cells are unclear. Adaptable gene circuits could enable practical applications in the life sciences and health care [22] . For example, finely tunable mammalian gene expression control systems could precisely relate protein levels to function, or could enable novel approaches to gene therapy. Most commonly, mammalian gene expression is tuned by gene expression systems. They consist of a regulator whose control over the expression of a target gene depends on the inducer level in the growth medium. For example, synthetic transactivator-based Tet-On/Off [23] and similar [24] systems have been widely utilized for gene expression control [25] . Yet, synthetic transactivators contain virus-derived activation domains [26] that can be toxic to mammalian cells [27] , interfering with normal cell physiology, and compromising the reliable assessment of gene function [28] . Repressor-based gene expression systems, such as the T-REx [29] and LacI systems [30] , avoid this problem as they lack viral activation domains. Yet, repressor-based systems can have sigmoidal dose response and highly variable gene expression at intermediate levels of induction [31] , making it difficult to bring all cells uniformly to defined intermediate levels of induction. These limitations create an unmet need to develop novel strategies for precise mammalian gene expression control [32] , [33] . One alternative, the ProteoTuner system [34] , relies on post-translational regulation—but requires fusing a destabilization domain to the gene of interest, which is not guaranteed to function seamlessly for all genes. We have previously developed a new, negative feedback based ‘linearizer’ gene circuit in yeast ( Fig. 1a ) with two attractive features: linear dependence of average gene expression on extracellular inducer concentration and uniform gene expression (low variability) across the cell population at all induction levels [35] . These characteristics arose as negative feedback-adjusted repressor protein expression to a level that was just enough to repress its own gene. A subsequent increase of inducer concentration allowed new protein synthesis, but only up to the level capable to overcome the sequestering effect of additional inducer. Consequently, the repressor level became proportional to the inducer concentration. Moreover, the expression of an additional gene from an identical promoter also depended linearly on the level of inducer [35] . 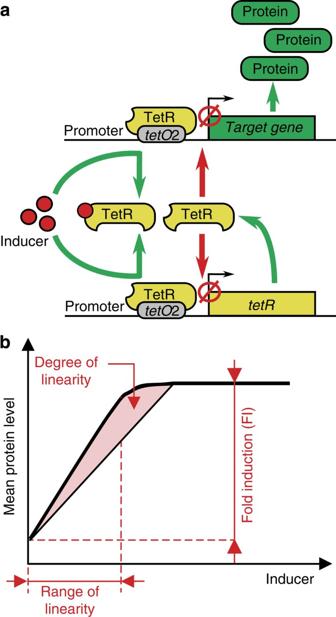Figure 1: Linearizer gene circuits and their performance characteristics. (a) A linearizer gene circuit consists of the TetR repressor and an arbitrary target gene, both controlled by the same promoter. In the absence of inducer (tetracycline or its derivatives), the TetR protein binds totetO2site(s) and physically blocks transcription from both promoters (red arrows). If inducer is added to the growth medium, it diffuses into cells and binds TetR, which dissociates from thetetO2sites (green arrows). Protein levels start to increase (green arrows) until TetR synthesis exceeds inducer influx and TetR blocks both promoters once again. (b) Performance metrics of linearizer gene circuits based on the dose-response curve, defined as the average gene expression versus the inducer level (thick black line). The fold induction is the ratio of maximal and minimal (background) expression. The range of linearity covers the inducer concentrations where dose response appears linear. The degree of linearity measures the straightness of dose response between two inducer concentrations by the L1-norm (based on the shaded area). In addition, gene expression variability is measured by the coefficient of variation (CV, not shown). Figure 1: Linearizer gene circuits and their performance characteristics. ( a ) A linearizer gene circuit consists of the TetR repressor and an arbitrary target gene, both controlled by the same promoter. In the absence of inducer (tetracycline or its derivatives), the TetR protein binds to tetO2 site(s) and physically blocks transcription from both promoters (red arrows). If inducer is added to the growth medium, it diffuses into cells and binds TetR, which dissociates from the tetO2 sites (green arrows). Protein levels start to increase (green arrows) until TetR synthesis exceeds inducer influx and TetR blocks both promoters once again. ( b ) Performance metrics of linearizer gene circuits based on the dose-response curve, defined as the average gene expression versus the inducer level (thick black line). The fold induction is the ratio of maximal and minimal (background) expression. The range of linearity covers the inducer concentrations where dose response appears linear. The degree of linearity measures the straightness of dose response between two inducer concentrations by the L1-norm (based on the shaded area). In addition, gene expression variability is measured by the coefficient of variation (CV, not shown). Full size image We hypothesized that these beneficial properties of the linearizer system could also be reproduced in mammalian cells using an identical circuit design. This is a challenging, yet rewarding, goal as no inducible mammalian systems exist for linearly dose-dependent tuning of gene expression. Based on this rationale, we set out to create a novel mammalian gene expression system for linearly tunable and uniform gene expression across the cell population. If successful, this effort should lead to greatly improved gene expression control, while revealing crucial steps applicable for moving synthetic gene circuits from yeast into mammalian cells. Performance metrics Synthetic gene circuits are built for predefined purposes, for example, to function as switches, logical gates or oscillators. To measure how well they fulfil these functions, performance metrics are needed. Possible performance metrics for linearizer gene circuits are ( Fig. 1b ): (i) the fold induction defined as the ratio of expression levels in the fully induced state (maximum expression) versus the fully repressed state (background expression); (ii) the range of linearity defined as the inducer concentration range where linearity holds; (iii) the coefficient of variation that measures the non-genetic variability of gene expression in the cell population [36] and (iv) the degree of linearity that evaluates the straightness of the dose response between two inducer concentrations, using parametric linear regression ( R 2 ) or the L1-norm [35] . The latter metric estimates the deviation of the measured dose dependence from a perfectly linear relationship, and falls within the [0... 0.5] range, with lower values indicating better linearity [35] . We applied these metrics to evaluate the performance of mammalian linearizer gene circuits. Importantly, the metrics are not entirely independent of each other. For example, measuring the degree of linearity requires some reasonable fold induction ( Fig. 1b ). The naïve prototype is non-functional in mammalian cells To facilitate troubleshooting, we first approached the problem of gene circuit transfer naïvely, using the design and components of the simplest yeast-based linearizer. In yeast, the gene circuit with fewest components that still had linear dose response and low noise was a fluorescent TetR::yEGFP fusion that could repress its own promoter [35] . To mimic this design, we built mammalian prototype TG1 ( Fig. 2a ) by expressing the bifunctional tetR::eGFP gene from pCMV-2xtetO, the Cytomegalovirus pCMV promoter [37] modified with two tetO2 sites downstream of the TATA box [29] in the widely used human breast adenocarcinoma MCF-7 cell line [38] . As in yeast, we expected tetR::eGFP self-repression to depend on the inducer concentration in the growth medium. 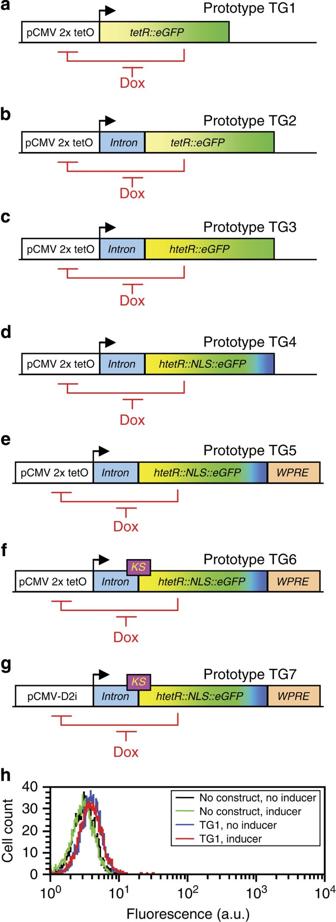Figure 2: Initial deficiency of expression and subsequent linearizer prototypes. (a) Mammalian linearizer prototype TG1, naïvely constructed based on a bifunctional repressor–reporter fusiontetR::eGFPfrom the original yeast circuit. (b) Prototype TG2, with an intron sequence introduced upstream oftetR::eGFP. (c) Prototype TG3, with the human codon-optimizedhtetR::eGFPgene. (d) Prototype TG4, with a NLS added betweenhtetRandeGFP. (e) Prototype TG5, with the WPRE sequence introduced into the 3′ UTR of the mRNA. (f) Prototype TG6, with the Kozak sequence (KS) introduced in the beginning of thehtetR::NLS::eGFPgene. (g) Prototype TG7, using the novel pCMV-D2i promoter. (h) Gene expression distributions of MCF-7 cells stably expressing the chromosomally integrated prototype TG1 (see panelc) in 0 ng ml−1doxycycline (blue) and 250 ng ml−1doxycycline (red), relative to controls (black and green). Figure 2: Initial deficiency of expression and subsequent linearizer prototypes. ( a ) Mammalian linearizer prototype TG1, naïvely constructed based on a bifunctional repressor–reporter fusion tetR::eGFP from the original yeast circuit. ( b ) Prototype TG2, with an intron sequence introduced upstream of tetR::eGFP . ( c ) Prototype TG3, with the human codon-optimized htetR::eGFP gene. ( d ) Prototype TG4, with a NLS added between htetR and eGFP . ( e ) Prototype TG5, with the WPRE sequence introduced into the 3′ UTR of the mRNA. ( f ) Prototype TG6, with the Kozak sequence (KS) introduced in the beginning of the htetR::NLS::eGFP gene. ( g ) Prototype TG7, using the novel pCMV-D2i promoter. ( h ) Gene expression distributions of MCF-7 cells stably expressing the chromosomally integrated prototype TG1 (see panel c ) in 0 ng ml −1 doxycycline (blue) and 250 ng ml −1 doxycycline (red), relative to controls (black and green). Full size image We measured the level of gene expression in repressed and fully induced conditions (at 0 and 250 ng ml −1 doxycycline, respectively) by flow cytometry in cells harbouring the TG1 circuit stably integrated into the genome. In all clones the fold induction was marginal, and maximum fluorescence was indistinguishable from the autofluorescence of untransfected MCF-7 cells ( Fig. 2h ). Considering that pCMV-2xtetO is a strong promoter [29] , we suspected that poor fold induction was owing to inappropriate expression of the tetR::eGFP fusion, supported by previous evidence for suboptimal tetR expression in mammalian cells [39] , [40] . We also observed that the dose response of reporter gene expression in the T-REx system (incorporating the original prokaryotic tetR gene without feedback, Supplementary Fig. S1c ) had a very short plateau, followed by an upslope at relatively low inducer concentrations. This is a known hallmark of compromised TetR expression in gene expression systems without feedback [41] . Computational modelling suggests optimization strategy As mentioned above, measuring the degree of linearity of a gene circuit’s dose response requires some reasonable fold induction ( Fig. 1b ). To understand how we could improve tetR::eGFP expression and rescue fold induction, we adapted an earlier computational model of the linearizer gene circuit [35] ( Fig. 3a ), modifying its parameters to reflect possible differences between yeast and mammalian cells ( Supplementary Note 1 ). The model still produced a linear relationship between the inducer concentration and TetR::EGFP expression in the rising portion of the dose–response curve ( Fig. 3b ). Next, we varied the parameters of the adapted model systematically to determine their individual effect on fold induction ( Fig. 4a–d ). The simulated dose responses indicated that fold induction should be improvable through changes increasing tetR::eGFP expression and function, specifically (i) increasing the transcription rate ( m , Fig. 4a ); (ii) increasing the translation rate ( p , Fig. 4b ); (iii) decreasing messenger RNA degradation rate ( μ , Fig. 4c ); (iv) or increasing the repressor-DNA-binding rate ( r , Fig. 4d ). 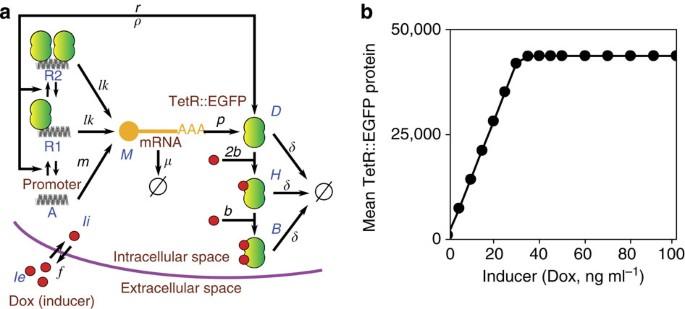Figure 3: Computational model and simulated dose response of the single-gene linearizer circuit. (a) Schematic representation of all chemical species, rates and reactions in the computational model. (b) Simulated mean oftetR::eGFPgene expression at different levels of inducer (Ie, doxycycline concentration, 0 to 100 ng ml−1). Figure 3: Computational model and simulated dose response of the single-gene linearizer circuit. ( a ) Schematic representation of all chemical species, rates and reactions in the computational model. ( b ) Simulated mean of tetR::eGFP gene expression at different levels of inducer ( I e , doxycycline concentration, 0 to 100 ng ml −1 ). 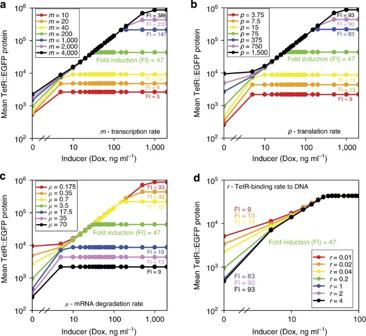Figure 4: The effect of parameter changes on the dose response of mean TetR::EGFP protein levels. Green curves represent nominal values of the parameters in the simulations. Each parameter was varied 5, 10 and 20 times up and down from the nominal value to investigate how it affects fold induction. Simulated inducer (Ie, doxycycline concentration) levels were between 0 and 1000, ng ml−1. (a) Increasing the transcription rate (m) improves fold induction. (b) Increasing the translation rate (p) improves fold induction. (c) Decreasing the mRNA degradation rate (μ) improves fold induction. (d) Increasing the TetR-DNA-binding rate (r) lowers minimum expression, while leaving the maximum expression unaffected, overall improving fold induction. Full size image Figure 4: The effect of parameter changes on the dose response of mean TetR::EGFP protein levels. Green curves represent nominal values of the parameters in the simulations. Each parameter was varied 5, 10 and 20 times up and down from the nominal value to investigate how it affects fold induction. Simulated inducer ( I e , doxycycline concentration) levels were between 0 and 1000, ng ml −1 . ( a ) Increasing the transcription rate ( m ) improves fold induction. ( b ) Increasing the translation rate ( p ) improves fold induction. ( c ) Decreasing the mRNA degradation rate ( μ ) improves fold induction. ( d ) Increasing the TetR-DNA-binding rate ( r ) lowers minimum expression, while leaving the maximum expression unaffected, overall improving fold induction. Full size image Following the suggestions from the model, we developed a three-stage strategy for restoring the function of the mammalian linearizer. First, at Stage 1 we planned to improve the efficiency of tetR::eGFP expression while minimizing background expression, to elevate fold induction. A summary of the changes applied to achieve this and the corresponding computational model parameters are listed in Supplementary Table S1 . A sufficiently large fold induction should allow testing the degree of linearity and level of noise at Stage 2. Finally, a target gene controlled by the same promoter could be introduced at Stage 3 to determine if linear dose response and gene expression uniformity would transfer to additional genes as they did in yeast. Intron insertion and codon optimization We reasoned that tetR::eGFP expression was suboptimal because the gene was ill-adapted to its mammalian host cells. Considering that pCMV-2xtetO is a strong promoter [29] , we decided to first concentrate our effort on improving translation ( p ) and mRNA stability ( μ ) of tetR::eGFP as suggested by the model. Seeking clues for gene circuit optimization, we looked for mammalian gene features less common in lower eukaryotes. One such feature is intron density [42] . Coincidentally, intron introduction into genes can increase their expression in mammalian cells [43] , [44] . The exact mechanism of this effect is not fully understood, but it is believed to be related to the enhancement of mRNA maturation and extranuclear transport by intron splicing [45] , [46] . This would increase mature mRNA levels, mimicking a decrease in the mRNA degradation rate μ in the computational model ( Fig. 4c ). Importantly, the same optimization was applied to tetR in the commercial T-REx system to improve its expression in mammalian cells. Considering all of the above, we introduced the rabbit β-globin intron II sequence [47] into the 5′-untranslated region (5′ UTR) of the yeast-derived tetR::eGFP sequence, obtaining prototype TG2 ( Fig. 2b ). We confirmed by reverse transcription PCR (RT-PCR) that the intron was properly spliced out from the mRNA, and the tetR::eGFP coding sequence was intact (data not shown). Another feature distinguishing mammalian and yeast gene sequences is synonymous codon usage bias. Adapting the codon bias to the host cell can improve heterologous gene expression in mammalian cells by improving translation efficiency [48] . Thus, we developed prototype TG3 ( Fig. 2c ) from prototype TG2 by rebuilding the repressor–reporter fusion from the mammalian codon-optimized variants of tetR ( htetR ) and eGFP genes [23] , [49] , with the aim of improving the translation rate p as suggested by the model ( Fig. 4b ). To test the effect of these changes, we transiently transfected all three prototypes into MCF-7 cells and measured their fluorescence level after 2 days of incubation in saturating inducer concentrations ( Fig. 5a ). The TG3 prototype had the strongest maximal expression (median fluorescence level of 466 a.u. in transfected cells) compared with TG1 (76 a.u.) and TG2 (269 a.u. ), respectively. This confirmed that the first pair of modifications improved htetR::eGFP expression. 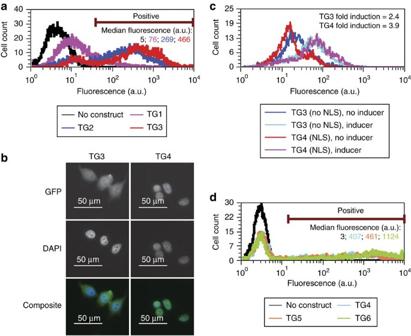Figure 5: Improving fold induction in prototypes TG2–TG6. (a) Gene expression distributions of MCF-7 cells transiently nucleofected with plasmids harbouring prototypes TG1, TG2 and TG3 in saturating concentration of inducer (1000, ng ml−1anhydrotetracycline). Median fluorescence was calculated for the cells carrying plasmid DNA. For control cells lacking plasmid DNA, the same statistics was calculated based on the entire population. (b) Fluorescent images of MCF-7 cells harbouring genome-integrated prototypes TG3 (no NLS, panels on the left) and TG4 (with NLS, panels on the right). EGFP fluorescence overlaid with 4',6-diamidino-2-phenylindole (DAPI) nuclear staining shows preferentially nuclear localization of TetR::NLS::eGFP in prototype TG4 compared with prototype TG3. The scale bar represents 50 μm. (c) Gene expression distributions of MCF-7 cells stably expressing genome-integrated prototypes TG3 and TG4 in 0 ng ml−1doxycycline (blue and red) and in 250 ng ml−1doxycycline (cyan and magenta), indicating the corresponding fold induction. (d) Gene expression distributions of MCF-7 cells transiently nucleofected with plasmids harbouring prototypes TG4, TG5 and TG6 in saturating inducer concentration (250 ng ml−1doxycycline). Median statistics was calculated as in (a). Figure 5: Improving fold induction in prototypes TG2–TG6. ( a ) Gene expression distributions of MCF-7 cells transiently nucleofected with plasmids harbouring prototypes TG1, TG2 and TG3 in saturating concentration of inducer (1000, ng ml −1 anhydrotetracycline). Median fluorescence was calculated for the cells carrying plasmid DNA. For control cells lacking plasmid DNA, the same statistics was calculated based on the entire population. ( b ) Fluorescent images of MCF-7 cells harbouring genome-integrated prototypes TG3 (no NLS, panels on the left) and TG4 (with NLS, panels on the right). EGFP fluorescence overlaid with 4',6-diamidino-2-phenylindole (DAPI) nuclear staining shows preferentially nuclear localization of TetR::NLS::eGFP in prototype TG4 compared with prototype TG3. The scale bar represents 50 μm. ( c ) Gene expression distributions of MCF-7 cells stably expressing genome-integrated prototypes TG3 and TG4 in 0 ng ml −1 doxycycline (blue and red) and in 250 ng ml −1 doxycycline (cyan and magenta), indicating the corresponding fold induction. ( d ) Gene expression distributions of MCF-7 cells transiently nucleofected with plasmids harbouring prototypes TG4, TG5 and TG6 in saturating inducer concentration (250 ng ml −1 doxycycline). Median statistics was calculated as in ( a ). Full size image Introducing a nuclear localization sequence The computational model indicated that gene expression increase from altering mRNA content and translation rate occurred at the expense of increased background expression ( Fig. 4b ). However, the model also suggested a remedy, indicating that increasing the repressor-DNA-binding rate r could compensate by lowering background expression while leaving the maximum expression unaltered ( Fig. 4d ). As direct improvement of repressor-DNA-binding affinity may require screening a large number of TetR mutants without a guarantee to find a variant with higher affinity, we decided to address this indirectly by introducing a nuclear localization sequence (NLS) into the tetR::eGFP coding sequence. While the addition of the NLS should not improve repressor-DNA-binding affinity directly, it should increase nuclear repressor protein concentration. This amounts to altering the effective binding rate of TetR::EGFP to tetO 2 sites in the promoter, mimicking an increase of the parameter r in the computational model. To test this, we introduced the simian virus 40 large-T-antigen NLS [50] into the middle of the TetR::EGFP protein, obtaining prototype TG4 ( Fig. 2d ). This should increase the effective binding rate of TetR::EGFP to the promoter by boosting the nuclear concentration of the repressor. Indeed, the NLS sequence caused preferential translocation of the TetR::NLS::EGFP protein into the nucleus in TG4 compared with the TG3 prototype ( Fig. 5b ) in bulk-selected MCF-7 cells stably expressing the genome-integrated TG3 and TG4 prototypes. Flow cytometry measurements in the absence and at saturating concentration of doxycycline (250 ng ml −1 ) indicated that prototype TG4 had higher fold induction than TG3 (3.9 and 2.4, respectively), confirming the computational predictions on gene circuit performance ( Fig. 5c ). Further changes in primary transcript sequence We surveyed the literature seeking additional modifications that could mimic the decrease in mRNA degradation rate μ suggested by the computational model. We found evidence that a particular sequence, the Woodchuck hepatitis virus post-transcriptional regulatory element (WPRE), boosted heterologous gene expression in mammalian cells [51] when placed in the 3′ UTR, presumably by enhanced mRNA polyadenylation, stabilization and extranuclear export. To test this possibility, we developed the TG5 prototype by introducing the WPRE into the 3′ UTR of the htetR::NLS::eGFP transcript ( Fig. 2e ). Further, to optimize the translation rate p as suggested by the model, we built prototype TG6 ( Fig. 2f and Supplementary Fig. S2 ) by converting the region around the ATG translation start codon to the consensus Kozak sequence, known to improve heterologous gene expression by enhancing translation in mammalian cells [52] . We tested how these changes influenced htetR::NLS::eGFP expression by transiently transfecting MCF-7 cells with the TG4, TG5 and TG6 prototypes using equal amounts of plasmid DNA (1 μg). Flow cytometry measurements after 2 days indicated a moderate improvement due to the WPRE sequence, while the Kozak sequence caused a dramatic gene expression increase ( Fig. 5d ; median fluorescence levels of 1,124, 461 and 407 a.u. for TG6, TG5 and TG4, respectively). Screening a novel library of TetR-repressible promoters The modifications applied so far in prototypes TG1–TG6 most likely altered cellular mRNA content, translation and protein localization. At the same time, the transcription rate m remained unoptimized in earlier prototypes, despite computational predictions of its strong effect on fold induction ( Fig. 4a ). One way to optimize m would be to create novel promoter variants and replace the pCMV-2xtetO promoter, originally created by inserting two tetO2 sites [29] between the TATA box and the Initiator (Inr) motif of the widely used parental wild-type pCMV promoter [37] ( Fig. 6a ). To accommodate the two tetO2 sites, the Inr motif was moved 54 bp downstream from its original position relative to the TATA box in the pCMV-2xtetO promoter [29] ( Fig. 6a ). We suspected that Inr displacement might have lowered maximum expression of the pCMV-2xtetO promoter, as in the wild-type pCMV promoter Inr was a transcription start site (TSS) crucial for efficient transcription [53] . To test this, we created a new promoter (pCMV-dInr), moving the Inr motif to exactly the same distance from the TATA box as in the pCMV-2xtetO promoter, but replacing the two tetO 2 sites with scrambled nucleotide sequences ( Supplementary Fig. S3a and Supplementary Note 2 ). Comparing eGFP expression from the wild-type pCMV, pCMV-2xtetO and pCMV-dInr promoters ( Supplementary Fig. S3b ) in transiently transfected MCF-7 cells, we found that the latter two promoters (with displaced Inr motifs) had significantly lower eGFP expression than the wild-type pCMV promoter ( Supplementary Fig. S3c ). In addition, we confirmed by RT–PCR (data not shown) that Inr ceased to be a TSS in pCMV-2xtetO, further confirming the suboptimality of the pCMV-2xtetO promoter structure. 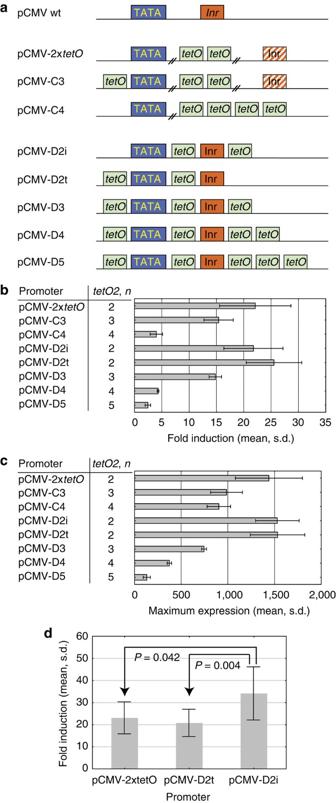Figure 6: A library of novel TetR-repressible promoters. (a) A schematic representation of wild-type pCMV, pCMV-2xtetO (Invitrogen) and two sets of novel TetR-repressible promoters with different numbers and positions oftetO2sites and with (pCMV-D2i, pCMV-D2t, pCMV-D3, pCMV-D4 and pCMV-D5) or without (pCMV-C3 and pCMV-C4) wild-type distance between the TATA box and the Inr motif. (b) Fold induction (mean±s.d.,n=5) in MCF-7 cells bulk transfected and stably expressing genome-integrated prototypes with the newly engineered promoters from (a). (c) Maximum expression (mean±s.d.,n=5, a.u., at 250 ng ml−1doxycycline) in the same MCF-7 cells as in (b). (d) Difference in fold induction between sets of clonal MCF-7 cell lines stably expressing TG prototypes based on the pCMV-2xtetO (mean±s.d.,n=7), pCMV-D2t (mean±s.d.,n=12) and pCMV-D2i (mean±s.d.,s=12) promoters (analysis of variance, overallP=0.003, followed by a Tukey HSD test: pCMV-D2i versus pCMV-2xtetO,P=0.042; pCMV-D2i versus pCMV-D2t,P=0.004). Figure 6: A library of novel TetR-repressible promoters. ( a ) A schematic representation of wild-type pCMV, pCMV-2xtetO (Invitrogen) and two sets of novel TetR-repressible promoters with different numbers and positions of tetO2 sites and with (pCMV-D2i, pCMV-D2t, pCMV-D3, pCMV-D4 and pCMV-D5) or without (pCMV-C3 and pCMV-C4) wild-type distance between the TATA box and the Inr motif. ( b ) Fold induction (mean±s.d., n =5) in MCF-7 cells bulk transfected and stably expressing genome-integrated prototypes with the newly engineered promoters from ( a ). ( c ) Maximum expression (mean±s.d., n =5, a.u., at 250 ng ml −1 doxycycline) in the same MCF-7 cells as in ( b ). ( d ) Difference in fold induction between sets of clonal MCF-7 cell lines stably expressing TG prototypes based on the pCMV-2xtetO (mean±s.d., n =7), pCMV-D2t (mean±s.d., n =12) and pCMV-D2i (mean±s.d., s =12) promoters (analysis of variance, overall P =0.003, followed by a Tukey HSD test: pCMV-D2i versus pCMV-2xtetO, P =0.042; pCMV-D2i versus pCMV-D2t, P =0.004). Full size image In addition to these ambiguities regarding the Inr sequence, there was no clear justification for the number and position of the tetO2 sites in the pCMV-2xtetO promoter. This is important because increasing the number of tetO2 sites could lower background expression in yeast [54] , raising another possibility to improve fold induction. Considering these uncertainties about the pCMV-2xtetO promoter structure and the computational suggestion to improve fold induction by increasing transcription efficiency ( Fig. 4a ), we set out to generate a library of newly synthesized promoters ( Supplementary Note 2 ), which could be screened for fold induction improvements. First, to determine how the number and position of additional tetO2 sites may affect fold induction in the context of the already characterized pCMV-2xtetO promoter, we inserted one or two additional tetO2 sites either upstream ( Fig. 6a , pCMV-C3) or downstream ( Fig. 6a , pCMV-C4) of the TATA box, regardless of the position of the Inr motif. Second, to determine whether restoring the wild-type position of the Inr motif relative to the TATA box increased maximum expression, while also reducing background expression depending on the number of tetO2 sites, we developed another set of promoters ( Fig. 6a ; pCMV-D2i, pCMV-D2t, pCMV-D3, pCMV-D4 and pCMV-D5) by introducing increasing numbers of tetO2 sites into the wild-type pCMV, spaced such that they left the relative position of the TATA box and Inr motifs intact. We tested the full set of novel promoters replacing the pCMV-2xtetO promoter with each of the eight reengineered promoter versions in the context of the TG6 prototype. This resulted in eight new intermediate prototypes that we transformed into MCF-7 cells. For each promoter variant, we selected cells in bulk to obtain polyclonal populations stably expressing the chromosomally integrated prototype and then measured by flow cytometry the background and maximum expression of the selected populations in 0 and 250 ng ml −1 doxycycline, respectively. Contrary to expectations, we found that fold induction and maximum expression generally decreased with the number of tetO2 sites in the promoter ( Fig. 6b ). In fact, the pCMV-2xtetO, pCMV-D2i and pCMV-D2t promoters with only two tetO2 sites conferred the highest fold induction (22.1±6.5, 21.8±5.4 and 25.5±5.1, respectively). In addition, these promoters also had the highest maximum expression among all gene circuit variants tested so far ( Fig. 6c ), and therefore we selected them for in-depth assessment. Next, we studied a set of clonal MCF-7 cell lines with stably genome-integrated constructs using the three promoters selected by preliminary screening. We expanded individual clones for each prototype (7 clones for the pCMV-2xtetO promoter, 12 clones for the pCMV-D2t promoter and 12 clones for the pCMV-D2i promoter) and assessed their fluorescence in both repressed and fully induced conditions. Flow cytometry measurements indicated that the pCMV-D2i promoter gave higher fold induction (34.0±12.0) than either of the pCMV-2xtetO and pCMV-D2t promoters ( Fig. 6d ; 22.9±7.2; P =0.042 and 20.6±6.2; P =0.004 respectively, based on analysis of variance). However, the maximal expression of these promoters did not differ significantly ( Fig. 6c and Supplementary Fig. S4 ), indicating that, at least in our settings, the pCMV-D2i promoter had optimal fold induction because of lower background expression rather than higher maximum expression. The promoter screen concluded Stage 1, throughout which fold induction had gradually improved, from negligible induction in the naïvely built TG1 prototype to 46-fold induction in the best clones expressing the TG7 prototype ( Supplementary Fig. S5 ), approaching the yeast linearizer’s performance [35] . The computational model guided these alterations causing gradual fold-change improvements. Finally, we selected the circuit with the pCMV-D2i promoter as the TG7 prototype ( Fig. 2g ) for further testing at Stage 2, owing to its highest fold induction among all tested prototypes ( Fig. 6d ). Linear dose response of gene expression in prototype TG7 To start assessing further performance characteristics at Stage 2, we concentrated on the dose response of a clonal MCF-7 cell line stably expressing the chromosomally integrated prototype TG7. Flow cytometry measurements at increasing inducer concentrations (0–25 ng ml −1 doxycycline) after 5 days of induction revealed a nearly linear dose response ( Fig. 7a , R 2 =0.99, L1-norm=4.0 × 10 −2 ) up to ~71% (6 ng ml −1 doxycycline) of the maximum expression ( Supplementary Fig. S6a ). In addition, the gene expression distributions were remarkably narrow ( Fig. 7b ), barring a few non-reacting cells, indicating uniform, linearly tunable gene expression over most inducer concentrations ( Fig. 7c ). These findings echo the performance of the yeast linearizer [35] , confirming its successful transfer from yeast to mammalian cells. 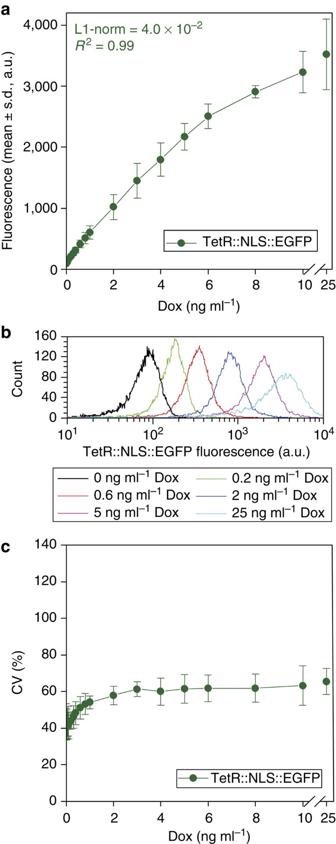Figure 7: Selection and assessment of prototype TG7. (a) Dose–response curve averaged for three independent assessments of MCF-7 cells stably expressing the genome-integrated prototype TG7 at increasing concentrations of doxycycline inducer (mean±s.d.). (b) Representative gene expression distributions of MCF-7 cells stably expressing the genome-integrated prototype TG7 at different levels of induction. (c) Variability of gene expression (coefficient of variation (CV)) averaged for three independent assessments of MCF-7 cells stably expressing genome-integrated prototype TG7 at increasing concentrations of doxycycline inducer (mean±s.d.). Figure 7: Selection and assessment of prototype TG7. ( a ) Dose–response curve averaged for three independent assessments of MCF-7 cells stably expressing the genome-integrated prototype TG7 at increasing concentrations of doxycycline inducer (mean±s.d.). ( b ) Representative gene expression distributions of MCF-7 cells stably expressing the genome-integrated prototype TG7 at different levels of induction. ( c ) Variability of gene expression (coefficient of variation (CV)) averaged for three independent assessments of MCF-7 cells stably expressing genome-integrated prototype TG7 at increasing concentrations of doxycycline inducer (mean±s.d.). Full size image Linearized regulation of a second target gene Finally, at Stage 3, we tested if dose–response linearity and gene expression uniformity can be transferred to another gene over a regulatory cascade as in yeast [35] . Thus, we introduced into the circuit the red fluorescent reporter mCherry , controlled by the same pCMV-D2i promoter and containing the same translational regulatory elements as the htetR::NLS::eGFP gene ( Fig. 8a ). 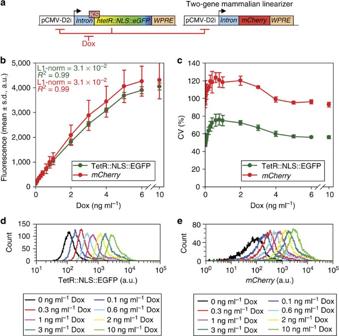Figure 8: Two-gene mammalian linearizer system. (a) Two-gene mammalian linearizer based on the TG7 prototype driving the expression of the fluorescent reporter genemCherry. (b) Dose–response curves ofhtetR::NLS::eGFPandmCherryexpression averaged for three independent measurements of MCF-7 cells stably expressing genome-integrated two-gene linearizer system at increasing concentrations of doxycycline inducer (mean±s.d.). (c) Variability (coefficient of variation (CV)) of gene expression forhtetR::NLS::eGFPandmCherrygenes measured as described for panel (b) (mean±s.d.). (d) Representative distributions of hTetR::NLS::EGFP measured by flow cytometry for the same cells as in panels (b) and (c). (e) Representative distributions ofmCherrymeasured by flow cytometry for the same cells as in panels (b) and (c). Figure 8: Two-gene mammalian linearizer system. ( a ) Two-gene mammalian linearizer based on the TG7 prototype driving the expression of the fluorescent reporter gene mCherry . ( b ) Dose–response curves of htetR::NLS::eGFP and mCherry expression averaged for three independent measurements of MCF-7 cells stably expressing genome-integrated two-gene linearizer system at increasing concentrations of doxycycline inducer (mean±s.d.). ( c ) Variability (coefficient of variation (CV)) of gene expression for htetR::NLS::eGFP and mCherry genes measured as described for panel ( b ) (mean±s.d.). ( d ) Representative distributions of hTetR::NLS::EGFP measured by flow cytometry for the same cells as in panels ( b ) and ( c ). ( e ) Representative distributions of mCherry measured by flow cytometry for the same cells as in panels ( b ) and ( c ). Full size image Flow cytometry measurements of an MCF-7 clonal cell line stably expressing this genome-integrated two-colour linearizer after 5 days of induction at increasing concentrations of doxycycline (0–25 ng ml −1 ) indicated a high fold induction in both parts of the circuit (30.8 and 38.5 for the htetR::NLS::eGFP and mCherry genes, respectively). Both dose responses were nearly linear up to 60 and 63% of the maximum expression of htetR::NLS::eGFP ( R 2 =0.99, L1-norm=3.1 × 10 −2 ) and mCherry ( R 2 =0.99, L1-norm=3.1 × 10 −2 ), respectively ( Fig. 8b and Supplementary Fig. S6b ), in contrast with the higher L1-norm values for the gene expression system without feedback ( Supplementary Fig. S6c ). The dose responses of average htetR::NLS::eGFP and mCherry expression were highly correlated ( Supplementary Fig. S6d ; Pearson correlation coefficient r =0.999, P <0.0001). Finally, gene expression distributions at different levels of induction were almost uniformly narrow ( Fig. 8c–e ) over the range of inducer concentrations. These findings demonstrate that this new mammalian gene expression system can impart dose–response linearity and gene expression uniformity to another arbitrary gene of choice, making gene expression precisely tunable. We achieved linearly inducer-dependent gene expression control and low gene expression variability in mammalian cells using a negative feedback-based gene circuit design identical to the one in yeast. These results confirm the adaptability of the yeast linearizer to mammalian cells without introducing any extra design features, solely by systematically optimizing parts responsible for efficient gene expression and protein localization. These two processes are at the heart of any synthetic gene circuit that employs regulators to control the expression of a target gene. Gene circuits will not function if a constituent gene is not expressed, or if a regulator lacks activity. Consequently, the steps we described should be relevant to transfer any synthetic gene circuit from microbes into mammalian cells. Even for gene circuits with more complex dynamics (such as bistable systems or oscillators), our strategy should enable adjustments to regain function lost in transfer across organisms. While some of these modifications were known to improve gene expression, their combined effect had not been tested quantitatively—especially in the context of synthetic gene networks, where the effects of modifications can interact in non-trivial manner, creating unpredictable behavior [54] . Overall, the novel parts we developed should greatly improve the performance of already existing mammalian gene constructs. For example, as TetR is widely used in mammalian synthetic biology [29] , [55] , our optimization steps can directly benefit other gene circuits employing this repressor, including T-REx. Compared with the existing T-REx gene expression system [29] , the main advantage of our design consists in allowing consistently precise and uniform gene expression control across a wide induction range, especially at intermediate levels of induction. For example, negative feedback-based systems such as prototype TG7 ( Fig. 2g ) or the two-gene linearizer ( Fig. 8a ) had very low L1-norm values (<0.1) for almost the entire rising portion of their dose–response curves (up to 70–80% of saturation, Supplementary Fig. S6a,b ), indicating linearity in that region. By contrast, the feedback-devoid T-REx system ( Supplementary Fig. S1a–d ) started from higher L1-norm values and continued to rise, with the exception of an intermediate portion ( Supplementary Fig. S6c ), indicating significant deviations from linearity. Moreover, contrary to the Tet-On/Off system [23] , the mammalian linearizer does not require a viral activation domain with toxic effects in mammalian cells that could be mistakenly attributed to the studied transgene [56] . Besides its advantages, the mammalian linearizer system also has some limitations that should be considered for practical usage. Owing to negative feedback regulation, it is expected to have somewhat higher background expression compared with systems based on repressor (T-REx) or transactivator (Tet-On) genes without feedback. This can limit the usage of the linearizer system for regulating strongly toxic genes. One way to decrease background expression in linearizer system could be to introduce a second repressor protein (such as LacI) or translational repression using the siRNA machinery [12] . We are currently working on implementing these improved linearizers with decreased background expression. Our results support the ‘abstraction principle’ in synthetic biology, illustrating how the different parts of a biological circuit can be optimized for better functionality in new biological settings, while leaving the overall design of the system intact. They also suggest the possibility to implement a synthetic biology pipeline, in which circuits are designed in silico , tested and characterized in lower eukaryotes (benefiting from their relatively easy genetic modification) and finally reimplemented and optimized for functionality in mammalian settings for practical usage. For example, the mammalian linearizer could be utilized in advanced vectors for highly needed [32] , [33] , precisely controlled gene expression in individualized gene therapy. This promising direction for treating genetic disorders and cancer could benefit from precisely tuning the expression of genes with narrow therapeutic window, such as rhodopsin [57] , according the patient’s condition and disease progression [22] , [32] , [33] . Moreover, linearizers could tune the expression of specific genes to reveal their effect on development, immune response or nervous system response. Finally, precisely tunable gene expression circuits and their constituent parts can be building blocks for more complex mammalian synthetic gene systems [58] , fostering progress in mammalian synthetic biology. Construction of plasmids The plasmids used in this study were constructed using the pcDNA4/TO and pcDNA6/TR plasmids from the T-REx system (Invitrogen, Carlsbad, CA) and the pDN-G1TGt yeast plasmid carrying the original tetR::eGFP gene. The oligonucleotides we used can be found in Supplementary Table S2 , while the detailed description of plasmid construction can be found in the Supplementary Methods . Cell lines and transfection MCF-7 (human breast adenocarcinoma cell line) and HEK 293 (human embryonic kidney cell line) were obtained from the American Type Culture Collection. MCF-7 and HEK 293 cell lines were maintained in RPMI 1640 and DMEM (Mediatech, Manassas, VA) media, respectively, each supplemented with 5% certified tetracycline-free fetal bovine serum (Clontech, Mountain View, CA). Cells were cultured at 37 °C, saturated with 5% CO 2 . For dose–response experiments, growth media were supplemented with different concentrations of doxycycline hydrochloride (Acros Organics, Geel, Belgium) and incubated with the inducer for 24–48 h (transiently transfected cells) or 120 h (stably expressing clones). Plasmid DNA into the cells was introduced using the Amaxa Nucleofector device (Lonza, Walkersville, MD), according to manufacturer protocol, using 5–10 × 10 6 cells, 1–5 μg of plasmid DNA, Solution V and program P-20. In transient transfection experiments, cells grew for 1–2 days before assessing them by flow cytometry. Plasmid DNA was linearized to obtain cell lines with stably genome-integrated gene circuits and cells were then selected using Zeocin (1000 μg ml −1 ) or Blasticidin (6 μg ml −1 ) drugs (Invitrogen) for 2–3 weeks. For lentivirus bulk infection, virions were packaged into the HEK 293 cell line and then used for infection of the target cells following the manufacturer’s protocol for the Lentiphos HT system and packaging plasmid mix (Clontech). Target MCF-7 cells were then selected using 2 μg ml −1 of Puromycin (Clontech) for 3 weeks. Flow cytometry and cell sorting Before flow cytometry, cells were trypsinized and resuspended in fresh media. Then cells were either read on a BD FACScan flow cytometer (BD Biosciences, San Jose, CA) using the 488-nm argon excitation laser and 530/30 emission filter (EGFP) or read/sorted on a BD FACSAria II (BD Biosciences) using the 488-nm blue excitation laser and 530/30 emission filter for EGFP and the 561-nm yellow-green excitation laser and 610/20 emission filter for mCherry . At least 5,000–6,000 cells were typically collected. Control experiments showed lack of significant spillover between the EGFP and mCherry channels in two-colour flow cytometry experiments ( Supplementary Fig. S7 ). Fluorescence microscopy For fluorescence microscopy, cells were grown on poly- D -Lysine-coated coverslips for 2 days and fixed with 4% paraformaldehyde (Electron Microscopy Sciences, Hatfield, PA) for 30 min. The coverslips were washed twice with PBS for 5 min and stained with 4',6-diamidino-2-phenylindole (1 μg ml −1 ) for 1 min. Images were acquired on a Nikon TE2000-E inverted fluorescence microscope (Nikon, Melville, NY) equipped with a CoolSNAP HQ [2] camera (Photometrics, Tucson, AZ), using a Nikon Plan Fluor 40 × /1.30 oil objective and B-2E/C filter (EX 465–495, DM 505 and BA 515–555 nm) for EGFP and a UV-2E/C filter (EX 340-380, DM 400 and BA 435–485 nm) for 4',6-diamidino-2-phenylindole (both from Nikon). Composite images with scale bars were prepared in NIS Elements (Nikon). Finally, all images were cropped and brightened uniformly in Adobe Photoshop (Adobe Systems, San Jose, CA). Reverse transcription PCR Total mRNA was isolated from the cells using the Qiagen RNEasy Mini Kit (Qiagen, Germantown, MD). Reverse transcription was performed using the GoScript™ Reverse Transcription System (Promega, Madison, WI), according to the manufacturer’s protocol. The complementary DNA of interest was then amplified using the primers: CMV-TSS+75-f, CMV-TSS-f and BGH-close-r (see Supplementary Table S2 for oligonucleotide sequences). Data processing and statistical analysis Flow cytometry data were analysed with FCS Express 3 (De Novo Software, Los Angeles, CA) and/or the flowCore package [59] in the R Project for Statistical Computing 2.13.1. Forward-scatter and side-scatter gates were used to minimize variation due to cell size, and a fluorescence-based gate was imposed to eliminate cells lacking gene circuits. One-way analysis of variance and post-hoc Tukey HSD test in STATISTICA 9.1 (StatSoft Inc., Tulsa, OK) were used for statistical comparison of clonal cell lines with different promoters. Only inducible cell sublines (fold induction ≥2) derived from the clonal populations with at least 90% of expressing cells and without multiple plasmid integrations (double peaks) were selected for analysis. We assessed linearity using the L1-norm [35] that varies from 0 (perfectly linear) to 0.5 (least linear). To determine the ranges of linearity for prototype TG7 ( Fig. 2g ), the two-gene mammalian linearizer ( Fig. 8a ) and the T-REx system ( Supplementary Fig. S1a ), we calculated the L1-norm for increasing ranges of inducer concentration starting from 0 ng ml −1 of doxycycline up to the maximum concentration used in the experiments ( Supplementary Fig. S6a–c ). Dose-response curves with <4 data points were not considered for L1-norm estimation. For each inducer dose range, we obtained the L1-norm in three steps: (i) we rescaled the relevant inducer concentrations and fluorescence values to the [0…1] range; (ii) we interpolated this rescaled dose-response curve using the function interp1 (piecewise cubic Hermite interpolating polynomial) from the signal package in the R Project for Statistical Computing 2.13.1 ( http://www.r-project.org/ ); (iii) we calculated and reported the L1-norm as the area enclosed by the rescaled dose-response curve and a straight line connecting the coordinates (0,0) to (1,1), using the trapz function from the caTools package in R. In addition to calculating the L1-norm, we also performed simple parametric linear regression to calculate R 2 as an alternative linearity metric using the R Project for Statistical Computing 2.13.1. Computational modelling and parameter scans We adapted an earlier computational model [35] changing parameters to account for biological differences between yeast and mammalian cells and implemented it in the software Dizzy [60] . We then used the computational model to study the effect of altering different parameters (the transcription rate m , the translation rate p , the mRNA degradation rate μ and the effective promoter-TetR::EGFP binding rate of r ) on the predicted values of fold induction, seeking clues on the biological processes that should be optimized first in linearizer circuit. The effect of these parameter scans was estimated for doxycycline concentrations ranging from 0 to 2000, ng ml −1 . The detailed description of the model, Dizzy code and parameters scans can be found in Supplementary Note 1 . A dditional information How to cite this article: Nevozhay, D. et al. Transferring a synthetic gene circuit from yeast to mammalian cells. Nat. Commun. 4:1451 doi: 10.1038/ncomms2471 (2013).